A halictid bee with sympatric solitary and eusocial nests offers evidence for Hamilton's rule The validity of Hamilton's rule has been confirmed among cooperative breeders where helping behaviour is transient; however, Hamilton's rule has not been validated among eusocial insects where helpers commit for life. Here we conduct a direct test of Hamilton's rule using field populations of Lasioglossum baleicum bees, which inhabit sympatric solitary and eusocial nests. Our results show that the indirect fitness of sterile first-brood workers is higher than the direct fitness of solitary first-brood females, and spring foundresses achieve a large direct fitness by having helpers. These fitness benefits are attributed to markedly higher larval survival rates in multiple-female nests, and intruding into an unrelated nest yields a moderate degree of direct fitness, but coexistence with unrelated females also increase overall brood survival. We discuss reasons why various types of cooperation are maintained in Lasioglossum baleicum with relation to that how a multiple-female nesting improves larval survival. Ever since Darwin pondered the question of how the worker traits of social insects are shaped by natural selection despite worker sterility [1] , the evolution of eusocial workers has remained one of the fundamental puzzles in evolutionary biology [2] , [3] . This question has been addressed by kin selection theory, which states that sterile workers compensate for decreased direct fitness by increasing indirect fitness through increasing direct reproduction of a related queen [4] . This principle has been referred to as Hamilton's rule ( br − c >0: here, r =relatedness between the donor and recipient, b =benefit to the recipient, and c =cost in direct fitness to the donor) [4] and is now applied to explain the evolution of generalized cooperation in many systems ranging from cell groups to human societies [2] , [3] . Although the validity of Hamilton's rule has been confirmed in several cooperative organisms where helping behaviour is transient (for example, cooperative microbes with cheats [5] or adoption of orphaned infants by squirrels [6] ), no direct test has been made in eusocial organisms. Only a small number of indirect tests of Hamilton's rule have been possible in eusocial insects because known eusocial species lack a sympatric solitary state that could serve as a control [7] , [8] . Therefore, in eusocial organisms, Hamilton's rule has not been directly tested in more than 50 years despite its fundamental importance. Cooperative halictid bees are suitable to study the evolution of sociality because their social organization varies widely over a geographic range, ranging from solitary behaviour in cold regions to eusocial behaviour in warm regions [9] , [10] , [11] , [12] , [13] . Morphological difference between the queens and workers is small or absent [13] . Importantly, recent investigations have revealed that solitary- and multiple-female nests occur in a single population of a halictid bee, Lasioglossum baleicum [14] , [15] . L. baleicum is a bivoltine bee that produces two broods per year, and multiple-female nests are found only during the second reproductive period [16] . Many colonies are constructed within a small area, producing nest aggregations [14] , [15] , [16] . Within each shallow nest (<10 cm below ground), a nest gallery containing several larval cells are constructed; each cell is provided with a pollen ball for rearing the larva [16] . In Sapporo, solitary females that have overwintered (F0) maintain nests and rear their first brood (F1) during the spring (early May to mid-June). After a short inactive period, a second brood is reared (F2) during mid-July to mid-August. No third reproduction has been observed most likely because the season is never long enough to complete a third reproduction [14] , [17] . The F2 females hibernate after mating and become new F0 foundresses in the following spring. The F1 broods contain males and females, and a fraction of the F1 females are inseminated [17] . During the second reproductive period, many nests contain multiple adult females; however, some nests are maintained by a single female [15] . This sympatric presence of solitary- and multiple-female nests in L. baleicum allows for Hamilton's rule to be directly tested in the field. We use 'multiple-female nest' for a nest containing multiple adult females and 'eusocial nest' for a nest that consists of a F0 female and F1 females. In bivoltine halictid bees, some F1 females seem to enter diapause without the second reproduction [18] . For example, L. baleicum populations inhabiting cold areas rear only a single brood [14] , [17] , suggesting that early diapause is an optional strategy for F1 females. In addition, adult females occasionally intrude into an unrelated nest [14] , [15] , [19] . In a previous study, bees nesting in a shady area did not produce a second brood [14] , which indicated that a F1 female can choose early diapause or intruding. Thus, at the start of the second reproductive period, F1 females can engage in the solitary nesting, eusocial nesting with the mother, intruding into another nest, or early diapause. 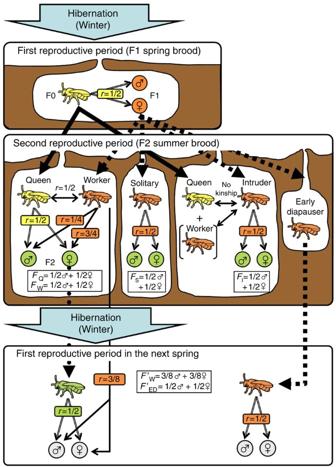Figure 1: Annual life cycle and options ofLasioglossum baleicumF1 females. The cycle begins with a solitary founding by an overwintered F0 female. Four possible options of a first-brood female (orange) are shown. The relatedness to offspring (r) and potential fitness of each strategy (F) are presented. Blue arrows represent winter. Thick dashed-arrows represent transfers to the next reproductive period, and thin solid arrows indicate relatedness between individuals. Figure 1 illustrates the annual life cycle of L. baleicum and how fitness would accrue for each of the four options above. Other than in early diapause, the fitness of each option can be measured by examining the content of the nest and genetic relationships among nest members at the end of the second reproductive period. Figure 1: Annual life cycle and options of Lasioglossum baleicum F1 females. The cycle begins with a solitary founding by an overwintered F0 female. Four possible options of a first-brood female (orange) are shown. The relatedness to offspring ( r ) and potential fitness of each strategy ( F ) are presented. Blue arrows represent winter. Thick dashed-arrows represent transfers to the next reproductive period, and thin solid arrows indicate relatedness between individuals. Full size image All else being equal, by comparing the fitness of solitary females with eusocial workers in a population, we can directly test Hamilton's rule in this study. It is possible that solitary females might be orphaned F1 workers that are forced into a deleterious condition; however, this possibility is not a problem for our purpose. Such an enforced condition may enable us to demonstrate the disadvantage of the solitary option, which is necessary for the upholding of Hamilton's rule. Comparing with more advanced bees (that is, bumblebee and honeybee), social halictid bees show little morphological differentiation between the F0 queens and F1 workers [13] , [20] . However, we carefully examined potential differences between females in the different social classes, because the potential equivalence between a solitary female and a eusocial worker is required to test Hamilton's rule. We compared fitness among the social classes of L. baleicum using two field populations over a 2-year period. All of the characteristics required to calculate fitness were measured using field and laboratory measurements, including microsatellite DNA analysis. A collected bee was classified into each of four social classes: queen, worker, orphaned worker, or intruder. We calculated the number of putative cooperative genes transmitted to the F2 generation (equivalent to fitness) for each adult female. By comparing the average fitness of each class, we examined whether Hamilton's rule is fulfilled for the worker bees, and how the indirect fitness benefits of worker bees arise from the increase in direct reproduction of the queen. On the basis of the results, we will discuss reasons why a helping behaviour evolves and how fitness benefits of helping behaviour arise in L. baleicum . Social organization of nests Each nest contained one-to-five adult females with the number of nests in each category (1–5 adult females) being 4, 3, 3, 4, 6 and 1, 12, 0, 0, 0 in 2009 and 2010, respectively. Detailed nest compositions are presented in Table 1 . Observations of morphological wear revealed that most multiple-female nests ( n =24) contained a single F0 female and 1-to-4 F1 females. In the remained nests, there were three types of colonies; nests consisted of unrelated F1 females that produced their own brood ( n =3), nests consisted of related F1 females ( n =1), and nests maintained by a single F1 female ( n =5). All of the F0 females were inseminated and had many yellow bodies in their ovaries, indicating they had laid eggs. In nests with an F0 female, most of the F1 females lacked yellow bodies (sterile); however, a small number did have yellow bodies (fertile). At five loci examined, all of the sterile F1 females had genotypes that matched the mother–daughter relationship with their F0 females; however, the fertile F1 females had at least one locus where the genotype(s) were incompatible with the mother–daughter relationship of the F0 female. These results indicate that the sterile F1 females were daughters of the F0 queen and that the fertile F1 females were unrelated intruders. Table 1 Nest composition of each nests in each year. Full size table Four multiple-female nests consisted only of F1 females. Three of the four nests consisted only of unrelated fertile-females (relatedness: 0.134±0.567, average±s.e.). The genotype analyses indicated that each female produced her own brood. In the remaining nest, the resident F1 females were full-sisters to each other (0.725±0.297). The genotype analyses showed that several F2 pupae in this nest are offspring of the resident F1 females, and the remaining F2 pupae could be assigned to an absent F0 female. Another female had been observed in this nest during the first reproductive period, confirming a loss of F0 females from the nest before the start of second reproductive period. These results showed that the F1 resident females in this nest were orphaned workers that produced their own brood. Genotypes of a small fraction of the F2 pupae in the eusocial nests with the intruders were compatible with the intruders, but not with the F0 female, indicating that the intruders produced their own brood. The average relatedness of the intruders to the progeny of the F0 female did not differ significantly from zero (0.0032±0.0161, average±s.e.). In nests without intruders, the F2 pupae had genotypes that were compatible with the queens, but not with the sterile F1 females, suggesting that all of the F2 pupae are the progeny of the queen. These findings enabled us to classify an adult female into each of the following five classes: a solitary female (S), a F0 queen (Q), a sterile daughter of the queen (eusocial worker; W), an orphaned fertile-worker (OW), and an intruder (I). Fitness comparisons among the female classes The used genotype matching method may overlook a small proportion of males resulting from workers because of genotype matching by chance [21] , [22] . The proportion of such males was estimated to be 13.5% at the P =0.05 significance level. However, as our analysis of yellow bodies showed that all of the eusocial workers were sterile, we could infer that all males were the queen's sons. Thus, we calculated the fitness of the F0 queens and F1 workers, under the assumption that all of the pupae other than those of the intruders were progeny of the queen. The fresh-weight population sex-investment ratios were not different from 0.5 (in 2009: 0.514, t =0.244, df=19, P =0.810; in 2010: 0.559, t =0.882, df=12, P =0.395, t -test), showing that we can neglect any concern for sex-ratio bias in further analyses. We estimated the fitness of each individual by assigning the pupae in a nest equally to each adult female. Number of pupae produced by a queen was assigned equally to the queens and eusocial workers. This treatment is set as a default, because there is no information for the difference in contribution among adult females to total brood production. In addition, as the larval survival rate of the multiple-female nests was much higher (ca. 9 times) than that of solitary nests (see below), the equal assignments would not be a cause of over- (or under-) estimation of fitness. Estimation of the mating frequency of the F0 females using the MATESOFT computer program [23] revealed that the queen mated once in 16 and 11 nests and twice in 4 and 2 nests in 2009 and 2010, respectively. However, sperm use was not biased from 1:1 in doubly mated queens (Wilcoxon signed-rank test, V =6, P =0.174). Thus, we used a relatedness value of 0.75 between a worker and an F2 female in the nests of singly mated queens and a value of 0.5 between them in nests with queens that mated twice. Relatedness between a worker and a brother was set to 0.25, and the relatedness between a mother and her daughters was set to 0.5. By weighting the assigned number of F2 pupae by the relatedness, we were able to estimate the number of gene copies that were transmitted from each adult female to the F2 generation. As a two-way ANOVA did not reveal any significant interaction between class and years ( P =0.793), we compared the average fitness among the classes for the pooled data over 2 years ( Fig. 2a ). Compared with class S, the fitness of class Q and class W are significantly high (Q versus S, P =0.003; W versus S, P =0.048; post-hoc test using Turkey–Kramer's method). The fitness of Q, W and OW did not significantly differ from each other (Q versus W, P =0.619; Q versus OW, P =0.535; W versus OW, P =0.872). The fitness of I was significantly lower than Q (I versus Q, P =0.001) but was not significantly lower than W (I versus W, P =0.112). The fitness of I was not statistically different from either S or OW (I versus S, P =0.664; I versus OW, P =0.999). The fitness was not different among the multiple-female nests with and without intruders ( Fig. 2b ). The results indicated that the average indirect fitness of a eusocial worker was higher than the direct fitness of a solitary female. Therefore, Hamilton's rule is upheld for eusocial workers. 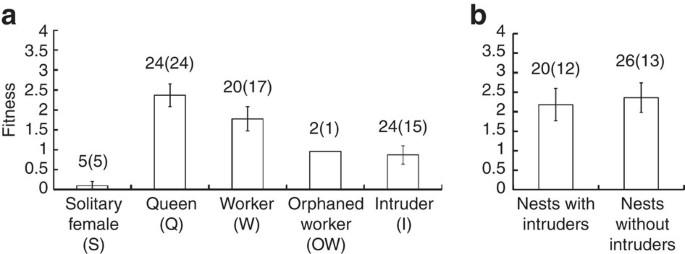Figure 2: Fitness as number of putative gene copies is transferred to second brood. (a) Average fitness of females in each cooperative class, and (b) the average fitness of a female in a nest with and without intruders. Numbers above bars indicate the number of individuals and nests (in parentheses). Bars show the average, and whiskers show the s.e. Statistical differences between classes are as follows: compared with solitary females (S), the fitness of queens (Q) and workers (W) are significantly higher (Q versus S,P=0.003; W versus S,P=0.048; a post-hoc test by the Turkey-Kramer's method). The fitness of Q, W and orphaned workers (OW) did not significantly differ from each other (Q versus W,P=0.619; Q versus OW,P=0.535; W versus OW,P=0.872). The fitness of intruders (I) was significantly lower than Q (I versus Q,P=0.001) but was not significantly lower than W (I versus W,P=0.112). Fitness of I was not statistically different from either S or OW (I versus S,P=0.664; I versus OW,P=0.999). Figure 2: Fitness as number of putative gene copies is transferred to second brood. ( a ) Average fitness of females in each cooperative class, and ( b ) the average fitness of a female in a nest with and without intruders. Numbers above bars indicate the number of individuals and nests (in parentheses). Bars show the average, and whiskers show the s.e. Statistical differences between classes are as follows: compared with solitary females (S), the fitness of queens (Q) and workers (W) are significantly higher (Q versus S, P =0.003; W versus S, P =0.048; a post-hoc test by the Turkey-Kramer's method). The fitness of Q, W and orphaned workers (OW) did not significantly differ from each other (Q versus W, P =0.619; Q versus OW, P =0.535; W versus OW, P =0.872). The fitness of intruders (I) was significantly lower than Q (I versus Q, P =0.001) but was not significantly lower than W (I versus W, P =0.112). Fitness of I was not statistically different from either S or OW (I versus S, P =0.664; I versus OW, P =0.999). Full size image Larval survival depending on social organization In one-way ANOVA testing of the pooled data, the number of cells produced per female was not different between the solitary and multiple-female nests ( Fig. 3a ). However, the rate of larval survival was markedly higher ( ∼ 9 times) in the multiple-female nests than in the solitary nests ( Fig. 3b ). Subsequently, the number of pupae produced per female was significantly larger in the multiple-female nests than in the solitary nests ( Fig. 3c ). These results show that the high fitness levels of the members of multiple-female nests are because of the high larval survival rates. The rate of larval survival was not different among the multiple-female nests with and without intruders (Mann–Whitney U -test, z =−0.850, P =0.932). 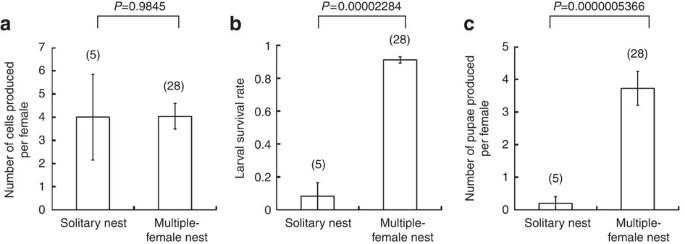Figure 3: Productivity measures of solitary- and multiple-female nests. (a) Number of cells produced per female. (b) Survival rates of larvae and (c) number of produced pupae per female. Average and s.e. are shown for each bar. Statistical significances using a one-way ANOVA are also shown. Figure 3: Productivity measures of solitary- and multiple-female nests. ( a ) Number of cells produced per female. ( b ) Survival rates of larvae and ( c ) number of produced pupae per female. Average and s.e. are shown for each bar. Statistical significances using a one-way ANOVA are also shown. Full size image Potential differences among the female classes The average head width of the F0 females was not different from the F1 females (Mann–Whitney U -test, U =333, P =0.585). All solitary females belonged to the F1 generation, and their average head width was not statistically different from eusocial F1 workers ( U =5, P =0.889), or from orphaned workers ( U =2, P =1.000) and intruders ( U =12, P =0.923). A fraction of the F1 females were inseminated (inseminated/the status has been confirmable/examined: solitary female, −/0/4; sterile F1 females, 0/6/12; orphaned workers, 0/2/2; intruders, 4/8/14). The obtained results did not show considerable differences among the female classes. In the orphaned and intruders' nests, the larval survival rate was not different from the eusocial nests (Fisher's exact probability test: for the orphaned nest, P =1.000; for the intruders' nest, P =1.000). This result indicates that multiple F1 females can successfully complete brood rearing without an F0 female and that the failure of the solitary females depends on being solitary as opposed to the absence of an F0 queen. The most important finding of this study is that the inclusive fitness of a eusocial worker was higher than that of a solitary female, with all else being equal. In addition, the inclusive fitness of a eusocial worker was indirectly generated from the progeny of the mother queen. The results demonstrate that the increased indirect-fitness compensates for the decreased direct-fitness of a eusocial worker. Thus, Hamilton's rule was satisfied in L. baleicum workers because of substantial indirect fitness gains. Several previous studies predicted increased fitness under multiple-female nesting compared with solitary nesting [7] , [8] . However, these studies were unable to perform direct fitness comparisons between solitary females and workers because all previously known eusocial species lack a directly comparable solitary state. Therefore, this study is the first report in which the satisfaction of Hamilton's rule has been shown using sympatric solitary and eusocial individuals in eusocial organisms. The satisfaction of Hamilton's rule has been shown in several cooperative, but not in eusocial, organisms [5] , [6] . In addition, positive kinship has been shown to precede helping behaviours in birds and mammals [24] , [25] . These results indicate that kin selection has a key role in the evolution of cooperation. The high fitness of members in multiple-female nests is attributed to high larval survival rates. The larval survival rate was ∼ 1/9 under solitary nesting ( Fig. 3b ). Unlike more advanced bees (for example, bumblebee and honeybee), there is little morphological differentiation of queens from the workers in halictid bees [13] , [20] . In this study, there was no difference in head width between the F0 queen and F1 workers. In addition, the presence of successful nests that consisted only of F1 females denies a possibility that the presence of an F0 queen is necessary for successful brood rearing. Thus, the failure of the solitary females is attributed to the solitary condition itself rather than the absence of an F0 queen. Queens also gained a large direct fitness, although the measured fitness is a part of the lifetime fitness of the F0 females. Thus, worker behaviour in L. baleicum would be beneficial to the queens and workers. The F0 females of halictid bees maintain their nests without helpers during the first reproductive period [12] , [13] , [16] , [19] . It has been suggested that the lack of lifetime monogamy may prevent the halictid bees from lifetime eusociality [26] . A fraction of F0 females mated twice. Thus, this view is worth examination in future studies of L. baleicum . Multiple-female nesting improves larval survival rates in L. baleicum . Multiple-female nests are likely to be more capable of defending against larvae predators. In both of the years studied, workers of the omnivorous ant, Tetramorium tsushimae , were found in the galleries of L. baleicum nests where most cells were empty [15] . In 2010, workers of this ant species were observed carrying a pupa out of an L. baleicum nest, which implies that this ant is a predator of L. baleicum larvae. Foraging T. tsushimae employ a mass recruitment system headed by a scout that searches for food items along the crevices of the ground's surface. The scout recruits numerous nestmates using a pheromone trail to tag a large food item [27] . As the larvae of L. baleicum are stored in shallow underground cells, the T. tsushimae scouts are highly likely to intrude directly into the larval cells. Although Lasioglossum bees frequently inspect larval cells after closing them [13] , [28] , the attendant bees would be unable to defend the larvae after a mass recruitment. Thus, inspector bees have to kill T. tsushimae scouts to defend larvae from predation. Unlike solitary bees, multiple-female nests can undertake more frequent inspections that increase the probability of the detection and removal of T. tsushimae scouts. A similar increase of productivity per female has been reported in an allodapine bee, and the predatory threat by ants has been suggested to result in the high mortality of solitary nests [29] . In L. baleicum , the start of multiple-female nesting corresponds with the increase in predatory activity [30] . All of evidence suggests that the cooperation of multiple females is effective against predation in halictid bees. The further experimental studies will highlight the selective pressure that promotes cooperation in L. baleicum . In L. baleicum , larval survival rates were drastically improved when number of adult females in a nest increase to more than one ( Fig. 3b ). The presence of F0 queen is not necessary for this success, because the nests that consisted only of F1 females showed high larval survival rates. Thus, our results demonstrate that cooperation itself is a crucial factor to increase fitness of a participated female. Our data also suggests that cell productivity per female slightly decreases with number of adult females in a nest ( Table 1 ). Although this point is important to discuss the optimal number of individuals in an already cooperative group, it is a different issue from the evolution of cooperation itself and will be examined in future studies. The eusocial F1 workers might benefit from avoidance of costs associated with independent nest founding (that is, head-start advantage [31] ). The independent founding allots more time for nest digging than retaining the mother nest. As temperature conditions at the study sites allow for two reproductive cycles in a summer [14] , time saving, using the head-start strategy, may be advantageous. In fact, nest inheritance is a hidden source of direct fitness in a polistine wasp [32] . However, although the solitary F1 females seem to have been transferred to the nest from the mother in the examined populations (see Methods), they could rear fewer pupae than the eusocial workers. Therefore, in L. baleicum , solitary nesting appears to be disadvantageous from the viewpoint of defence to predation irrespective of nest inheritance. One of the issues requiring further investigation is the occurrence of behaviours associated with relatively low fitness (that is, solitary nesting and intruding). As all of the solitary females were F1 females, it is possible that they have accidentally lost their F0 mother. As fitness was much lower under solitary nesting, this behaviour is not an independent strategy, but rather an enforced bad condition. In addition, all of the obtained results suggest that there was no difference in potential ability for nest maintenance between the solitary and the other class females. Therefore, this situation would enable us to test Hamilton's rule because the rule is satisfied only when the solitary option is disadvantageous. In L. baleicum , males have been produced in the F1 generation [17] ; however, only a part of the F1 females was inseminated in the study areas. The low insemination rate of the F1 generation is a normal condition in this species [17] . Although the solitary F1 females in this study might not be inseminated (insemination status was not confirmable for these individuals), the sole F2 male that survived in their nest has matched genotypes with the nest owners. This result did not reject a possibility of direct reproduction by the nest owner. In addition, the nest observation confirmed that solitary nest owner maintained their nests during the second reproductive period. None of the data indicated the presence of an F0 queen in the solitary nests during the second reproductive period. Direct reproduction of the orphaned workers also suggests that uninseminated F1 females can produce broods and that the disadvantageous choices of the solitary females might be a best of bad jobs. Direct reproduction by unrelated intruders has been reported in several bee species [19] , [33] , [34] . In our data, the intruders take their own share of direct reproduction; however, the members of the host nests obtained similar level fitness comparing with the eusocial nests without intruders ( Fig. 2b ). Thus, there is no net loss for members of the host nests of intruders. This situation suggests that there is little selection for efficient nest mate recognition, which allows this form of intruding to continue. In addition, L. baleicum nests in shady areas disappear in the second reproductive period in Sapporo probably because of a shortage of degree-day accumulation [14] . F1 females in such nests may become intruders rather than early diapausers (see below). In addition, solitary nesting can develop into a multiple-female state by receiving intruders into the nest. Thus, a solitary female may receive intruders as they may improve the survival rate of the brood. Indeed, seven multiple-female nests consisted of an F0 female and F1 intruders ( Table 1 ). Thus, in L. baleicum , a considerable proportion of nests consisted of only unrelated females. Wide variations in social organizations are usual in cooperative halictid bees [13] . It is interesting to study variation in social organization with relation to proximate mechanisms that promote cooperation in halictid bees. Of the four possible strategies of F1 females, this study did not measure the fitness of early diapausers. However, the fitness of the early diapausers seems to be lower than other strategies. Relatedness of an early diapauser or a eusocial worker to an individual of the next F1 generation (female or male) is 1/2 (=0.5) or 3/8 (=0.375), respectively ( Fig. 1 ). During hibernation, the survival rate of early diapausers can be assumed to be equal with the F2 females. In this case, if a eusocial worker can produce more than 1.33 (=0.5/0.375) F2 individuals, the worker behaviour is more advantageous than early diapause. A eusocial worker produced 4.300±0.549 F2 females (average±s.d., n =20), suggesting that the worker strategy is advantageous on average. Of course, F0 queens may produce a small number of early diapausers as a hedge bet for abnormally cold summers where the second reproduction cycle cannot be completed. The numbers of offspring produced by an intruder were not statistically different from the 1.33 threshold (1.438±0.387, n =20) but was still larger than the threshold. A solitary female could produce far less offspring than this threshold (0.200±0.200, n =5). However, if mortality during summer diapause is high, the early diapause may further be disadvantageous. Such a high mortality during the summer is expected because the foraging activity of the predator is high in the summer season [30] . In conclusion, early diapause seems to be disadvantageous in the studied populations on average. Study organism and field collection Halictid bees construct larval cells underground. Each cell contains a pollen ball on which the female lays a single egg. Many species are bivoltine in a year and multiple-female nests occur only after the second reproductive period [16] , [35] . By carefully excavating the nests at the end of a reproductive period, it is possible to determine the number of cells that were produced and number of pupae that were successfully reared. The sweat bee L. baleicum exhibits social polymorphism within a population [15] ; overwintered females (F0) usually produce two broods within a year (a spring brood (F1), and a summer brood (F2)). Many summer nests contain multiple adult females, and larval survival has been shown to correlate positively with the number of adult females in a nest [15] . Many colonies are constructed within a small area and results in nest aggregation [16] . We searched for nest aggregations in mid-May (start of the first reproductive period) in 2009 and 2010 at two sites in south-central Sapporo, Japan: the experimental forest of the Forestry and Forest Products Research Institute and Sapporo Experimental Forest of the Field Science Center for the Northern Biosphere, Hokkaido University. In early July (start of the second reproductive period), the individual bees of each nest were marked at two points on the thorax using a combination of seven colours made with a marker pen (PaintMarker; Mitsubishi, Japan). Using these marks, the number of adult bees in a nest was recorded. All of the nests were excavated in late August after the last larvae of the year had pupated. We conducted nest excavations in the early morning or late afternoon to avoid missing foraging bees. The contents of the cells were recorded as being male, female or empty. Adult females were dissected to confirm the presence of yellow bodies in their ovaries, which is evidence of egg laying. Insemination status of individuals was also recorded when we could identify the spermatheca. The degrees of wing and mandible wear were recorded for each adult to estimate her generation [16] . The specimens were genetically barcoded to identify species because other Lasioglossum species have been observed to cohabit with L. baleicum in nest aggregations [16] . One adult female per nest was subjected to mitochondrial DNA sequencing (1,152 bp of the CO–COII region, GenBank Accession No. AB299367 ) [14] to identify the species. The live weight of each F2 pupa was measured, and the population sex-investment ratio to females (females/(females+males)) was calculated based on the live weight to test a deviation from the 1:1 (=0.5) ratio statistically. Genetic analysis and determination of kinship Screening of 52 microsatellite loci for polymorphisms revealed 5 polymorphic loci, 4 of which have been previously described (LernC8, LernE6, LleuA52 and LoenE10) [36] , [37] , [38] and one (skb91a) was newly revealed in this study (forward: 5′-GTAACCCCTGGTCGCGAGTGCGA-3′, reverse: 5′-GATCTGCCTCTGGCGGGACCCA-3′; GenBank Accession No. AB627356 ). Each individual was genotyped for these loci using a genetic analyser (CEQ-8000, Beckman-Coulter). PCR conditions for the known loci were the same as those reported previously [36] , [37] , [38] whereas the conditions used for skb91a were the same as those used for LleuA52 (ref. 36 ). Kinship between any two individuals within a nest was determined by comparing genotypes between two individuals (genotype-matching analysis). As the assumed kinship is limited to the mother–offspring relationship in the second reproductive period, any incompatible genotypes (impossible allele(s) between the mother and her offspring) on at least one locus indicated that the examined pair is not a mother–offspring pair. Relatedness between individuals was estimated using the RELATEDNESS computer program (ver. 5.0.8) [39] . Adult females in a nest were first classified by generation (F0 or F1) based on the extent of wing and mandible wear [16] . Genotypes at each locus were compared for all possible F0–F1 pairs within a nest. As there were no nests with more than one F0 female, we considered an F1 female to be the daughter of the F0 female, if there were no incompatible marker loci. In several nests, number of adult females at the collection decreased from that during the nest observation period. If there were F2 pupae those genotypes did not match with any resident females, we estimated the genotype of the no-longer-present female from a genotype array of the offspring. Individual pupae were assigned to a female based on the following criteria: adult females with at least one incompatible locus with a pupa were removed from the candidate of mother; females that did not have any yellow bodies on the ovary were removed from the candidate of mother; when the above two criteria could not assign a pupa to a female, the pupa was assigned to one of the candidates by examining the relatedness of females to the pupa by considering the asymmetric relatedness in a haplodiploid organism. None of the eusocial F1 workers had yellow bodies, and thus, the third criterion was used to assign the pupae to either the F0 queen or an intruder. When a male showed matched genotypes with the F0 female at all loci, there is also a non-zero possibility that the male has been produced by a daughter of the F0 female. Although we checked for the presence of yellow bodies for each individual, the expected proportion of the overlooked worker reproduction was statistically estimated [21] , [22] . In addition, the mating frequency of the F0 female in a nest was estimated by examining the genotype array of her daughters using the MATESOFT computer program (ver. 1.0) [23] . We paid special attention to validate the mating number of females to avoid wrong diagnoses. When an F0 female was judged to mate multiple times, we validated that the diagnosis was not based on a 1–2-bp difference at a single locus, which might have been a misreading or amplification error [40] . When the diagnosis was based on such a difference, we re-checked the accuracy of the reading by loading both of the samples in the same capillary of the DNA analyser. In addition, we tested the possibility of amplification error by checking the readable pattern of the alleles. As most amplification errors yielded a short 'ghost' band by one microsatellite repeat [40] , we confirmed that the F0 female and her daughters showed clear banding patterns that did not show a large peak at the 'ghost' position. Estimation of fitness For each adult female, we calculated fitness as the number of copies of a putative cooperative-gene transmitted to the F2 generation. Fitness of an individual was estimated by weighting number of assigned F2 pupae by relatedness of the individual to them. For intruders and orphaned workers, we assigned their own brood. For a queen and her sterile F1 workers, we equally assigned F2 offspring of the queen to each related females. The equal assignment might be doubted because the indirect fitness of a worker arises from an increase in the queen's direct reproduction [3] . However, there is no data on reproduction by a single F0 female in the second reproductive period. In addition, we lack information for differences in the contribution of each female to total brood rearing in multiple-female nesting. Therefore, the equal assignment is justified as a default. When marked adults had disappeared from the nest before the nest digging ('Unknown' in Table 1 ), we averaged values of fitness in extreme cases (all unknowns were kin of the F0 queen or were intruders). We used theoretical relatedness instead of estimated relatedness in the calculations (that is, 0.5 for mother–offspring, 0.75 for full-sister, and 0.25 for brothers). In nests with a doubly-mated queen, relatedness was set to 0.5 for half-sisters because sperm use is not biased (see results section). Statistics The calculated fitness was averaged for each class, and the differences among the classes were examined using two-way ANOVA for class and year. When no interaction was detected between class and year, a single ANOVA on the pooled data over 2 years was conducted. As there are five classes, to correct for the statistical effects of multiple comparisons, differences between two classes were examined using a post-hoc test (Turkey–Kramer's method) [41] . Larval survival rates of the solitary and multiple-female nests were first compared using a two-way ANOVA before being compared using a single ANOVA after a confirmation of no significant interaction between the nest type and year. Differences in the fitness of adult females in host and non-host nests were examined using the Mann–Whitney U -test. Deviation of the population sex-investment ratio was statistically tested using the paired t -test. All of the statistical tests were conducted using R (ver. 2.9.2; R Development Core Team). Acccession codes: The sequence data have been deposited in the GenBank CoreNucleotide database under accession codes AB299367 and AB627356 . How to cite this article: Yagi, N. & Hasegawa, E. A halictid bee with sympatric solitary and eusocial nests offers evidence for Hamilton's rule. Nat. Commun. 3:939 doi: 10.1038/ncomms1939 (2012).